Skin thymic stromal lymphopoietin initiates Th2 responses through an orchestrated immune cascade Thymic stromal lymphopoietin (TSLP) has emerged as a key initiator in Th2 immune responses, but the TSLP-driven immune cascade leading to Th2 initiation remains to be delineated. Here, by dissecting the cellular network triggered by mouse skin TSLP in vivo , we uncover that TSLP-promoted IL-4 induction in CD4 + T cells in skin-draining lymph nodes is driven by an orchestrated ‘DC-T-Baso-T’ cascade, which represents a sequential cooperation of dendritic cells (DCs), CD4 + T cells and basophils. Moreover, we reveal that TSLP-activated DCs prime naive CD4 + T cells to produce IL-3 via OX40L signalling and demonstrate that the OX40L-IL-3 axis has a critical role in mediating basophil recruitment, CD4 + T-cell expansion and Th2 priming. These findings thus add novel insights into the cellular network and signal axis underlying the initiation of Th2 immune responses. Thymic stromal lymphopoietin (TSLP) is a short-chain four α-helical bundle type I cytokine, which is expressed mainly by epithelial cells in the skin, lung and intestine [1] . Studies in recent years have implicated TSLP as a master regulator of Th2 inflammatory responses in allergic diseases [2] , [3] . A link between TSLP and human atopic dermatitis (AD) was initially suggested following observations showing an increased expression of TSLP in the epidermis of AD skin, as well as that human TSLP-conditioned dendritic cells (DCs) induced Th2 development [4] . Using mouse models, our previous studies [5] and those of others [6] showed that induced expression of TSLP in mouse skin keratinocytes (KCs) triggers an AD-like syndrome, characterized by infiltration of CD4 + T cells and eosinophils, increased levels of Th2 cytokines and elevated serum IgE levels. Our studies further revealed that TSLP expression was regulated by nuclear receptors (that is, retinoid X receptors, retinoid acid receptors and vitamin D receptors) and found that topical treatment of mouse skin with the vitamin D3 low-calcemic analogue MC903 (known also as calcipotriol) induced TSLP expression in epidermal KCs, which subsequently generated an AD syndrome [7] , [8] . Furthermore, transgenic mice overexpressing TSLP in lung epithelial cells [9] were shown to develop a spontaneous asthmatic lung inflammation, and intradermal [10] or intranasal [11] delivery of TSLP induced tissue inflammation and Th2 cytokine production. However, although these studies established that TSLP was a key initiator of Th2 inflammatory responses, the underlying cellular and molecular mechanism remained still elusive. Numerous data (see reviews [3] , [12] and references therein) suggested that TSLP may act on various immune cells including DCs, T cells, NK cells, NKT cells, B cells, mast cells, eosinophils, basophils, as well as innate lymphoid cells [13] , but these data were based either on in vitro TSLP stimulation of a particular cell type or at a particular snapshot time of analyses, and therefore did not provide information on the immune cascade driven by TSLP within the tissue microenvironment. To achieve a better mechanistic understanding of TSLP-triggered immune responses, it is crucial to delineate the nature of key cellular factors and how they sequentially act and cross-talk in an in vivo context to initiate Th2 responses. Taking advantage of our established mouse experimental model to induce TSLP expression in epidermal KCs by topical treatment with MC903 (refs 7 , 8 ), we dissect here the immune cascade leading to Th2 initiation. Particularly, we focus on the initiation of IL-4 (the master regulator that promotes Th2 differentiation [14] ) in CD4 + T cells of skin-draining lymph nodes (LNs), where the T-cell priming could take place. We reveal that TSLP drives a ‘DC-T-Baso-T’ cellular cascade representing a sequential and orchestrated action of DCs, CD4 + T cells and basophils, which subsequently leads to IL-4 priming in CD4 + T cells. Importantly, we uncover that TSLP-activated DCs, through OX40L signalling, prime naive CD4 T cells to produce IL-3 and identify the critical role of TSLP (KCs)-OX40L (DCs)-IL-3 (CD4 T cells) axis in mediating basophil recruitment, CD4 + T-cell expansion and Th2 priming. Skin TSLP induces IL-4 priming in CD4 + T cells TSLP expression was induced in skin keratinocytes of wild-type (WT) Balb/c mice via MC903 (but not vehicle ETOH) treatment on ears every other day starting from day (D) 0 ( Fig. 1a ). As reported [7] , [8] , the TSLP expression was increased in treated ears ( Fig. 1b , left panel) but not in the ear-draining lymph nodes (EDLN) ( Fig. 1b , right panel). To investigate TSLP-triggered Th2 priming, we first analysed IL-4 expression in EDLN. MC903-induced IL-4 expression became evident at D5, which was barely detected at D3 ( Fig. 1c ). In contrast, there was no difference in IFNγ or IL-17 expression in EDLN of MC903- or ETOH-treated mice at D5 ( Supplementary Fig. S1 ), suggesting that MC903 selectively induces Th2 differentiation. Importantly, the IL-4 induction by MC903 was abolished in Tslp −/− mutant mice ( Fig. 1d ), demonstrating that TSLP was required for IL-4 expression in draining LNs. 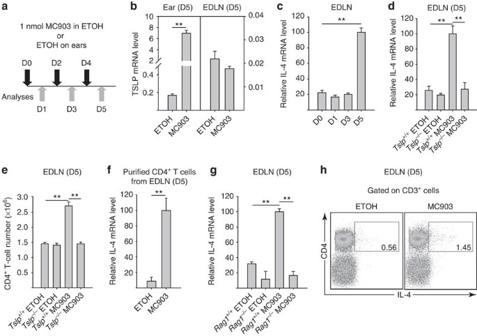Figure 1: Skin topical MC903 treatment induces TSLP-dependent Th2 priming in CD4+T cells in the skin-draining lymph nodes. (a) Experimental protocol. Mouse ears were topically treated with MC903 or ethanol (ETOH; as vehicle control) every other day from day (D) 0 to D4 and analysed at D1, D3 or D5. (b) TSLP mRNA level of ears and ear-draining lymph nodes (EDLN) from MC903- or ETOH-treated wildtype (WT) Balb/c mice at D5. (c) Relative IL-4 mRNA level in EDLN from MC903-treated WT Balb/c mice at D0, D1, D3 and D5. (d) MC903-induced IL-4 expression at D5 is abolished inTslp−/−mice. (e) CD4+T-cell number in EDLN of ETOH- or MC903-treatedTslp+/+andTslp−/−mice at D5. (f) Relative IL-4 mRNA level in purified CD4+T cells from EDLN of ETOH- or MC903-treated WT mice. (g) Relative IL-4 mRNA level in EDLN of ETOH- or MC903-treatedRag1+/+andRag1−/−mice. (h) Frequency of IL-4-producing CD4+T cells in EDLN from ETOH- or MC903-treated WT mice at D5. **P<0.005 (Student’st-test). Values are mean±s.e.m. (n≥3). Data are representative of three independent experiments with similar results. Figure 1: Skin topical MC903 treatment induces TSLP-dependent Th2 priming in CD4 + T cells in the skin-draining lymph nodes. ( a ) Experimental protocol. Mouse ears were topically treated with MC903 or ethanol (ETOH; as vehicle control) every other day from day (D) 0 to D4 and analysed at D1, D3 or D5. ( b ) TSLP mRNA level of ears and ear-draining lymph nodes (EDLN) from MC903- or ETOH-treated wildtype (WT) Balb/c mice at D5. ( c ) Relative IL-4 mRNA level in EDLN from MC903-treated WT Balb/c mice at D0, D1, D3 and D5. ( d ) MC903-induced IL-4 expression at D5 is abolished in Tslp −/− mice. ( e ) CD4 + T-cell number in EDLN of ETOH- or MC903-treated Tslp +/+ and Tslp −/− mice at D5. ( f ) Relative IL-4 mRNA level in purified CD4 + T cells from EDLN of ETOH- or MC903-treated WT mice. ( g ) Relative IL-4 mRNA level in EDLN of ETOH- or MC903-treated Rag1 +/+ and Rag1 −/− mice. ( h ) Frequency of IL-4-producing CD4 + T cells in EDLN from ETOH- or MC903-treated WT mice at D5. ** P <0.005 (Student’s t -test). Values are mean±s.e.m. ( n ≥3). Data are representative of three independent experiments with similar results. Full size image We next investigated whether TSLP-triggered IL-4 expression occurs in CD4 + T cells. Upon MC903 treatment, the total CD4 + T-cell number increased in EDLN of WT but not of Tslp −/− mice ( Fig. 1e ), and IL-4 expression was found to be induced in purified CD4 + T cells from EDLN of MC903-treated mice, when compared with ETOH-treated mice ( Fig. 1f ). Accordingly, TSLP-induced IL-4 expression was completely abolished in Rag1 −/− mice that lack mature T and B cells ( Fig. 1g ). Moreover, intracellular staining showed that IL-4 + cells were detected in the CD3 + CD4 + population ( Fig. 1h ), and their frequency was increased in EDLN from MC903-treated mice ( Fig. 1h ). Together, these results demonstrated that, upon MC903 topical treatment, skin-derived TSLP induced IL-4 expression in CD4 + T cells in the draining LNs. Dendritic cells are essential for the skin TSLP-induced IL-4 priming DCs are known to have a pivotal role in T-cell-mediated immunity including Th2 responses. Accumulation of DCs in EDLN was first examined at different time points upon MC903 treatment. An increase in CD11c + MHCII + cell number in EDLN became apparent at D3 ( Fig. 2a ) before IL-4 induction could be detected (see Fig. 1c ). To determine whether DCs are required for TSLP-triggered Th2 initiation, we made use of CD11c-DTR transgenic mice [15] in which CD11c hi DCs can be depleted by the administration of diphtheria toxin (DT). CD11c-DTR Tg/0 mice and their control littermates (CD11c-DTR 0/0 ) received an intraperitoneal ( i.p. ) injection of DT at D1 (thereafter called CD11c DEP mice and CD11c CT mice, respectively). When analysed one day later (that is, D0), a significant reduction of the CD11c hi MHCII + cells was observed in both ear dermis and EDLN of CD11c DEP mice ( Fig. 2b ). These mice were then treated with ETOH or MC903 at D0, D2 and D4 as indicated in Fig. 1a . Depletion of DCs did not affect the expression levels of skin TSLP induced by MC903 ( Fig. 2c ). However, IL-4 induction in EDLN ( Fig. 2d ), as well as in purified CD4 + T cells from EDLN ( Fig. 2e ), was abolished in MC903-treated CD11c DEP mice, indicating an essential role of DCs in TSLP-triggered IL-4 priming. Furthermore, we found that the number of CD4 + T cells increased in MC903-treated CD11c CT mice at D5 (as compared with ETOH treatment) but not in CD11c DEP mice ( Fig. 2f ). 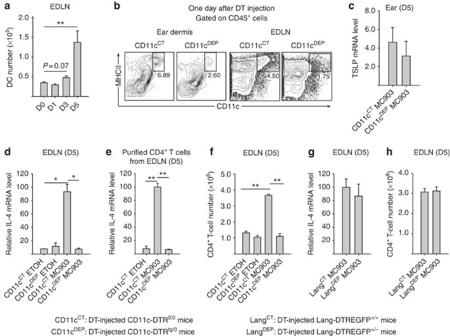Figure 2: CD11chidendritic cells are crucial for skin TSLP-promoted IL-4 priming. (a) Dendritic cell (DC; CD11c+MHCII+) number in ear-draining lymph nodes (EDLN) of MC903-treated wild-type (WT) Balb/c mice at D0, 1, 3 and 5. (b) Frequency of CD11c+MHCII+DCs in the ear dermis and EDLN of CD11cDEP(CD11chiDC-depleted mice; diphtheria toxin (DT)-injected CD11c-DTRtg/0mice) and CD11cCTcontrol (DT-injected CD11c-DTR0/0wildtype littermates) mice at one day after DT treatment. (c) No difference of TSLP mRNA level in MC903-treated ears from CD11cCTand CD11cDEPmice at D5. (d,e) Relative IL-4 mRNA level in EDLN (d) and in purified CD4+T cells from EDLN (e) from ETOH- or MC903-treated CD11cCTand CD11cDEPmice. (f) CD4+T-cell number in EDLN of MC903- or ETOH- treated CD11cCTand CD11cDEPmice at D5. (g) Relative IL-4 mRNA level in EDLN from LangDEP(Langerhans cell-depleted mice; DT-injected Lang-DTREGFP+/−mice) and LangCTcontrol mice (DT-injected Lang-DTREGFP+/+littermates), upon MC903 treatment at D5. (h) CD4+T-cell number in EDLN of MC903-treated LangCTand LangDEPmice at D5. *P<0.05, **P<0.005 (Student’st-test). Values are mean±s.e.m. (n=3). Data are representative of three independent experiments with similar results. Figure 2: CD11c hi dendritic cells are crucial for skin TSLP-promoted IL-4 priming. ( a ) Dendritic cell (DC; CD11c + MHCII + ) number in ear-draining lymph nodes (EDLN) of MC903-treated wild-type (WT) Balb/c mice at D0, 1, 3 and 5. ( b ) Frequency of CD11c + MHCII + DCs in the ear dermis and EDLN of CD11c DEP (CD11c hi DC-depleted mice; diphtheria toxin (DT)-injected CD11c-DTR tg/0 mice) and CD11c CT control (DT-injected CD11c-DTR 0/0 wildtype littermates) mice at one day after DT treatment. ( c ) No difference of TSLP mRNA level in MC903-treated ears from CD11c CT and CD11c DEP mice at D5. ( d , e ) Relative IL-4 mRNA level in EDLN ( d ) and in purified CD4 + T cells from EDLN ( e ) from ETOH- or MC903-treated CD11c CT and CD11c DEP mice. ( f ) CD4 + T-cell number in EDLN of MC903- or ETOH- treated CD11c CT and CD11c DEP mice at D5. ( g ) Relative IL-4 mRNA level in EDLN from Lang DEP (Langerhans cell-depleted mice; DT-injected Lang-DTREGFP +/− mice) and Lang CT control mice (DT-injected Lang-DTREGFP +/+ littermates), upon MC903 treatment at D5. ( h ) CD4 + T-cell number in EDLN of MC903-treated Lang CT and Lang DEP mice at D5. * P <0.05, ** P <0.005 (Student’s t -test). Values are mean±s.e.m. ( n =3). Data are representative of three independent experiments with similar results. Full size image We also examined whether epidermal Langerhans cells (LCs) could be implicated in TSLP-induced IL-4 priming. LCs were not depleted in the above CD11c DEP mice [16] . To deplete langerin + cells including epidermal LCs, we injected DT to Lang-DTREGFP +/− mice [17] (called thereafter Lang DEP mice). Interestingly, similar increases in IL-4 expression and CD4 + T-cell number in EDLN were observed in MC903-treated Lang DEP and Lang CT (DT-injected Lang-DTREGFP +/+ control littermates) ( Fig. 2g,h ), indicating that LCs were not implicated in TSLP-driven IL-4 induction in CD4 + T cells at D5. Basophils are required for TSLP-triggered IL-4 priming The role of basophils in Th2 cell differentiation in different models of allergy remains highly controversial (see reviews [18] , [19] and refs therein). To investigate their contribution in TSLP-induced Th2 priming, we first examined whether basophils were recruited into EDLN upon MC903 skin treatment. Flow cytometry analyses showed that basophils (identified as CD3 − B220 − CD49b + CD45 int FcεRIα + CD117 − Gr1 − ) [20] were barely detected in EDLN at D0, whereas their number was increased at D5 upon MC903 treatment ( Fig. 3a ). Kinetic analyses showed that such an increase started at D3 ( Fig. 3b ). MC903-induced basophil recruitment in EDLN was driven by TSLP, as it was completely abolished in Tslp −/− mice ( Fig. 3c ). 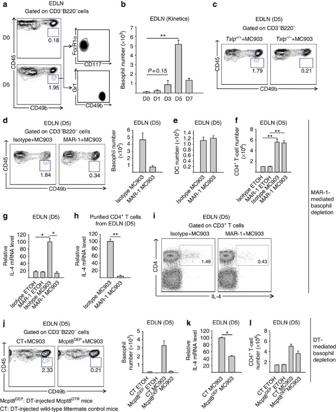Figure 3: Basophils are required for skin TSLP-promoted IL-4 priming in CD4+T cells. (a) Representative FACS plots of basophils in ear-draining lymph nodes (EDLN) of MC903-treated wild-type (WT) Balb/c mice at D0 and D5. Basophils in EDLN are gated as CD45intCD49b+cells in non-B non-T (CD3−B220−) population, which are characterized as FcεRI+CD117−Gr1−cells. (b) Basophil number in EDLN of MC903-treated WT Balb/c mice at D0, 1, 3, 5 and 7. (c) Frequency of basophils in EDLN of MC903-treatedTslp+/+andTslp−/−mice at D5. (d) Frequency and total number of basophils in EDLN of isotype or MAR-1 antibody (Ab)-injected WT mice, upon MC903 treatment at D5. (e) DC number in EDLN from isotype or MAR-1 Ab-injected WT mice, upon MC903 treatment at D5. (f) Total CD4+T-cell number in EDLN of isotype or MAR-1 Ab-injected WT upon ETOH or MC903 treatment at D5. (g) Relative IL-4 mRNA level in EDLN of isotype or MAR-1 Ab-injected WT mice upon MC903 or ETOH treatment at D5. (h) Relative IL-4 mRNA level in purified CD4+T cells from EDLN of isotype or MAR-1 Ab-injected WT mice upon MC903 treatment at D5. (i) Frequency of IL-4+CD4+T cells in EDLN of isotype or MAR-1 Ab-injected WT mice, upon MC903 treatment at D5. (j) Frequency and total number of basophils in EDLN of Mcpt8DEP(DT-injected Mcpt8DTRmice) and CT (DT-injected WT littermate control mice), upon MC903 treatment at D5. (k) Relative IL-4 mRNA level in EDLN of Mcpt8DEPand CT mice, upon MC903 treatment at D5. (l) Total CD4+T-cell number in EDLN of Mcpt8DEPand CT mice, upon MC903 treatment at D5. *P<0.05, **P<0.005 (student’st-test). Values are mean±s.e.m. (n=3). Data are representative of two or three independent experiments with similar results. Figure 3: Basophils are required for skin TSLP-promoted IL-4 priming in CD4 + T cells. ( a ) Representative FACS plots of basophils in ear-draining lymph nodes (EDLN) of MC903-treated wild-type (WT) Balb/c mice at D0 and D5. Basophils in EDLN are gated as CD45 int CD49b + cells in non-B non-T (CD3 − B220 − ) population, which are characterized as FcεRI + CD117 − Gr1 − cells. ( b ) Basophil number in EDLN of MC903-treated WT Balb/c mice at D0, 1, 3, 5 and 7. ( c ) Frequency of basophils in EDLN of MC903-treated Tslp +/+ and Tslp −/− mice at D5. ( d ) Frequency and total number of basophils in EDLN of isotype or MAR-1 antibody (Ab)-injected WT mice, upon MC903 treatment at D5. ( e ) DC number in EDLN from isotype or MAR-1 Ab-injected WT mice, upon MC903 treatment at D5. ( f ) Total CD4 + T-cell number in EDLN of isotype or MAR-1 Ab-injected WT upon ETOH or MC903 treatment at D5. ( g ) Relative IL-4 mRNA level in EDLN of isotype or MAR-1 Ab-injected WT mice upon MC903 or ETOH treatment at D5. ( h ) Relative IL-4 mRNA level in purified CD4 + T cells from EDLN of isotype or MAR-1 Ab-injected WT mice upon MC903 treatment at D5. ( i ) Frequency of IL-4 + CD4 + T cells in EDLN of isotype or MAR-1 Ab-injected WT mice, upon MC903 treatment at D5. ( j ) Frequency and total number of basophils in EDLN of Mcpt8 DEP (DT-injected Mcpt8 DTR mice) and CT (DT-injected WT littermate control mice), upon MC903 treatment at D5. ( k ) Relative IL-4 mRNA level in EDLN of Mcpt8 DEP and CT mice, upon MC903 treatment at D5. ( l ) Total CD4 + T-cell number in EDLN of Mcpt8 DEP and CT mice, upon MC903 treatment at D5. * P <0.05, ** P <0.005 (student’s t -test). Values are mean±s.e.m. ( n =3). Data are representative of two or three independent experiments with similar results. Full size image We next depleted basophils in WT mice via i.p. injection of an antibody (Ab) specific to FcεRIα (MAR-1) [21] , [22] , before MC903 treatment. Depletion of basophils was confirmed at D5 in EDLN from MAR-1-injected mice ( Fig. 3d ). Of note, the number of DCs at D5 was similarly increased in both isotype and MAR-1 Ab-injected mice upon MC903 treatment ( Fig. 3e ). In addition, the increase in CD4 + T-cell number was similar in EDLN from MAR-1- or isotype-injected mice ( Fig. 3f ), suggesting that, in contrast to DC depletion ( Fig. 2f ), basophil depletion did not affect CD4 + T-cell expansion. However, TSLP-triggered IL-4 expression in CD4 + T cells in EDLN was clearly decreased in MAR-1-injected mice ( Fig. 3g,h ). This was also confirmed by IL-4 intracellular staining ( Fig. 3i ). As recent studies have raised concerns about possible deleterious effects of MAR-1 on other cells than basophils [18] , such as mast cells [21] or subset of DCs [23] , particularly when high doses of MAR-1 were administrated [23] , we further performed experiments using two other depletion strategies, that is, Ba103 (antibody specific to CD200R3)-mediated basophil depletion [24] ( Supplementary Fig. S2a ) and DT-mediated basophil depletion in Mcpt8 DTR mice [22] ( Fig. 3j ). Both of these basophil depletions led to a significantly diminished IL-4 induction in CD4 + T cells upon MC903 treatment ( Fig. 3k and Supplementary Fig. S2c,d ), while the increase in CD4 + T-cell number was not altered by basophil depletion ( Fig. 3l and Supplementary Fig. S2b ). Thus, we concluded that basophils have an important role in priming CD4 + T cells to express IL-4, whereas they are dispensable for the expansion of CD4 + T cells. DCs and CD4 + T cells are required for basophil recruitment We then explored the cellular mechanism through which basophils are recruited into EDLN. Upon the depletion of DCs in CD11c DEP mice, TSLP-triggered basophil recruitment was abolished, as shown by decreases in both the frequency and total number of basophils ( Fig. 4a ), indicating that DCs were crucial for basophil recruitment into EDLN. 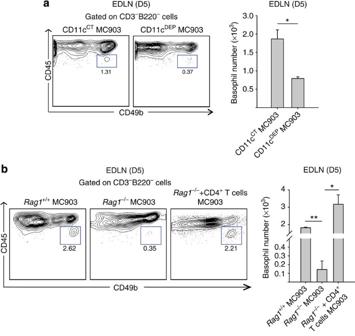Figure 4: DCs and CD4+T cells are required for TSLP-promoted basophil recruitment in skin-draining lymph nodes. (a) Frequency and total number of basophils in ear-draining lymph nodes (EDLN) of MC903-treated CD11cDEPand CD11cCTmice at D5. CD11cDEP, DT-injected CD11c-DTRtg/0mice; CD11cCT, DT-injected CD11c-DTR0/0WT control littermate mice. (b) Frequency and total number of basophils in EDLN of MC903-treatedRag1+/+,Rag1−/−and WT CD4+T-cell-reconstitutedRag1−/−mice at D5. *P<0.05, **P<0.01 (student’st-test). Values are mean±s.e.m. (n≥3). Data are representative of two independent experiments with similar results. Figure 4: DCs and CD4 + T cells are required for TSLP-promoted basophil recruitment in skin-draining lymph nodes. ( a ) Frequency and total number of basophils in ear-draining lymph nodes (EDLN) of MC903-treated CD11c DEP and CD11c CT mice at D5. CD11c DEP , DT-injected CD11c-DTR tg/0 mice; CD11c CT , DT-injected CD11c-DTR 0/0 WT control littermate mice. ( b ) Frequency and total number of basophils in EDLN of MC903-treated Rag1 +/+ , Rag1 −/− and WT CD4 + T-cell-reconstituted Rag1 −/− mice at D5. * P <0.05, ** P <0.01 (student’s t -test). Values are mean±s.e.m. ( n ≥3). Data are representative of two independent experiments with similar results. Full size image As DC depletion abolished CD4 + T-cell expansion ( Fig. 2f ), we next examined whether CD4 + T cells may have a role in recruiting basophils in EDLN. Upon MC903 treatment, basophil recruitment was abolished in Rag1 −/− mice but could be restored in these mice when reconstituted with WT CD4 + T cells ( Fig. 4b ). Together, these results indicated that TSLP-triggered basophil recruitment into the EDLN required both DCs and CD4 + T cells. TSLP-activated DCs trigger IL-3 expression by CD4 + T cells On the basis of the above results, we posited that the basophil recruitment could be mediated by factor(s) derived from DC-primed CD4 + T cells. As IL-3 derived from CD4 + T cells has been recently implicated in basophil recruitment to LNs in a helminth infection mouse model [25] , we examined whether IL-3 could be involved in TSLP-triggered basophil recruitment in EDLN. We first performed kinetic analyses of IL-3 expression upon MC903 treatment and found that IL-3 mRNAs were not detected at D0 or D1 but started to increase from D3 ( Fig. 5a ), which correlated well with basophil recruitment in EDLN (see Fig. 3b ). Interestingly, the IL-3 increase was detected earlier (at D3) than that of IL-4 (at D5) (compare Figs 1c and 5a ), indicating that IL-3 induction could precede IL-4 priming. 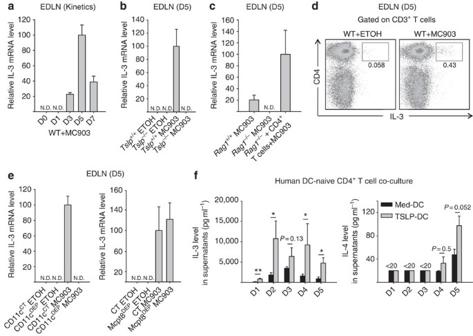Figure 5: TSLP-activated DCs induce IL-3 expression in CD4+T cells. (a) Relative IL-3 mRNA level in ear-draining lymph nodes (EDLN) from MC903-treated wild-type (WT) Balb/c mice at various time points, showing that the induction of IL-3 expression was detected as early as at D3 and peaked at D5. ND, not detected. (b) Relative IL-3 mRNA level in EDLN from ETOH- or MC903-treatedTslp+/+andTslp−/−mice at D5. (c) Relative IL-3 mRNA level in EDLN of MC903-treatedRag1+/+,Rag1−/−and WT CD4+T-cell-reconstitutedRag1−/−mice at D5. (d) Frequency of IL-3+CD4+T cells in EDLN from ETOH- or MC903-treated WT Balb/c mice at D5. (e) Relative IL-3 mRNA level in EDLN from MC903- or ETOH-treated CD11cDEPand CD11cCTmice (left panel), and from MC903-treated Mcpt8DEPand CT mice (right panel). (f) TSLP-conditioned human DCs (TSLP-DC) promote an earlier production of IL-3 than IL-4 by human naive CD4+T cells. Med-DC, medium-conditioned DCs. *P<0.05, **P<0.01 (Mann–Whitney test). Values are mean±s.e.m. (a–e,n=3;f,n=6). Data are representative of two independent experiments with similar results. Figure 5: TSLP-activated DCs induce IL-3 expression in CD4 + T cells. ( a ) Relative IL-3 mRNA level in ear-draining lymph nodes (EDLN) from MC903-treated wild-type (WT) Balb/c mice at various time points, showing that the induction of IL-3 expression was detected as early as at D3 and peaked at D5. ND, not detected. ( b ) Relative IL-3 mRNA level in EDLN from ETOH- or MC903-treated Tslp +/+ and Tslp −/− mice at D5. ( c ) Relative IL-3 mRNA level in EDLN of MC903-treated Rag1 +/+ , Rag1 −/− and WT CD4 + T-cell-reconstituted Rag1 −/− mice at D5. ( d ) Frequency of IL-3 + CD4 + T cells in EDLN from ETOH- or MC903-treated WT Balb/c mice at D5. ( e ) Relative IL-3 mRNA level in EDLN from MC903- or ETOH-treated CD11c DEP and CD11c CT mice (left panel), and from MC903-treated Mcpt8 DEP and CT mice (right panel). ( f ) TSLP-conditioned human DCs (TSLP-DC) promote an earlier production of IL-3 than IL-4 by human naive CD4 + T cells. Med-DC, medium-conditioned DCs. * P <0.05, ** P <0.01 (Mann–Whitney test). Values are mean±s.e.m. ( a – e , n =3; f , n =6). Data are representative of two independent experiments with similar results. Full size image Next, we showed that MC903-induced IL-3 expression was abolished in Tslp −/− mice ( Fig. 5b ). The induction of IL-3 was abrogated in MC903-treated Rag1 −/− mice, but adoptive transfer of WT CD4 + T cells fully restored IL-3 expression ( Fig. 5c ). In addition, intracellular staining showed that the frequency of IL-3 + CD4 + T cells was increased in EDLN upon MC903 treatment ( Fig. 5d ). These results demonstrated that TSLP triggers the IL-3 expression by CD4 + T cells. Furthermore, upon DC depletion, TSLP-triggered IL-3 expression in EDLN was totally abolished; in contrast, it was not affected by basophil depletion, thus indicating that, in TSLP-driven immune cascade, IL-3 expression by CD4 + T cells is downstream of DCs but not of basophils ( Fig. 5e ). We further sought to verify that TSLP-stimulated DCs trigger an early IL-3 expression in CD4 + T cells, by employing an in vitro human DC-naïve CD4 + T cell co-culture system [4] , [26] . Previous studies using this system have shown that DCs activated by TSLP could prime allogenic naive CD4 + T cells to produce more IL-4 after 6 or 7 days of co-culture [4] , [26] . By performing kinetic analyses, we found with interest that, upon the priming with TSLP-DC, naive CD4 + T cells produced an increased amount of IL-3 as early as after 1 day of co-culture ( Fig. 5f , left panel; compare TSLP-DC with medium(med)-conditioned DC); in contrast, the increase in IL-4 production began to be seen only after 5 days of co-culture ( Fig. 5f , right panel). Such a kinetic fits with the timing observed in vivo in our mouse model, both of which indicate that TSLP-activated DCs prime CD4 + T cells to produce IL-3 at a stage that precedes the initiation of IL-4 expression. IL-3 is crucial for basophil recruitment and IL-4 induction What could be the possible role of IL-3 in TSLP-triggered Th2 initiation process? We then applied MC903 topical treatment on Il3 −/− mice and found that these mice exhibited a decrease in basophil recruitment in EDLN, compared with MC903-treated WT mice ( Fig. 6a ). In addition, there was lesser increase in CD4 + T-cell number in EDLN ( Fig. 6b ) These data indicated that IL-3 had an important role in both basophil recruitment and CD4 + T-cell expansion in skin-draining LNs. RT–PCR analyses showed that TSLP-driven IL-4 expression in EDLN at D5 was significantly reduced in Il3 −/− mice ( Fig. 6c ). Moreover, intracellular staining showed a lower frequency of IL-4 + CD4 + T cells in MC903-treated Il3 −/− mice ( Fig. 6d ), indicating that IL-3 was required for TSLP-driven IL-4 induction in CD4 + T cells. 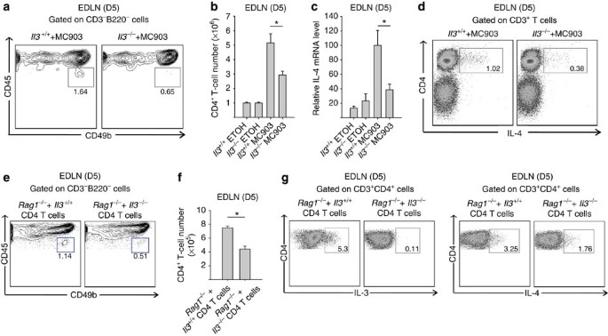Figure 6: IL-3 produced by CD4+T cells is required for basophil recruitment and for IL-4 priming in CD4+T cells. (a–d) Comparison of basophil frequency (a), CD4+T-cell number (b), IL-4 mRNA level (c) and IL-4+CD4+T-cell frequency (d) in EDLN of MC903-treatedIl3+/+andIl3−/−mice at D5. (e–g) Comparison of basophil frequency (e), CD4+T-cell number (f) and frequency of IL-3+CD4+(g; left panel) and IL-4+CD4+(g; right panel) T cells in EDLN of MC903-treatedRag1−/−mice reconstituted with CD4+T cells fromIl3+/+orIl3−/−mice. *P<0.05 (Student’st-test). Values are mean±s.e.m. (n≥3). Data are representative of two independent experiments with similar results. Figure 6: IL-3 produced by CD4 + T cells is required for basophil recruitment and for IL-4 priming in CD4 + T cells. ( a – d ) Comparison of basophil frequency ( a ), CD4 + T-cell number ( b ), IL-4 mRNA level ( c ) and IL-4 + CD4 + T-cell frequency ( d ) in EDLN of MC903-treated Il3 +/+ and Il3 −/− mice at D5. ( e – g ) Comparison of basophil frequency ( e ), CD4 + T-cell number ( f ) and frequency of IL-3 + CD4 + ( g ; left panel) and IL-4 + CD4 + ( g ; right panel) T cells in EDLN of MC903-treated Rag1 −/− mice reconstituted with CD4 + T cells from Il3 +/+ or Il3 −/− mice. * P <0.05 (Student’s t -test). Values are mean±s.e.m. ( n ≥3). Data are representative of two independent experiments with similar results. Full size image Furthermore, upon MC903 treatment, Rag1 −/− mice reconstituted with Il3 −/− CD4 + T cells showed a decrease in basophil recruitment ( Fig. 6e ), CD4 + T-cell number ( Fig. 6f ), as well as IL-4 expression ( Fig. 6g ), when compared with Rag1 −/− mice reconstituted of WT CD4 + T cells. These results thus demonstrated that IL-3 produced by CD4 + T cells is crucial for recruiting basophils into skin-draining LNs and for inducing IL-4 expression in CD4 + T cells. The OX40L-OX40 signalling promotes IL-3 expression We then explored which molecules derived from TSLP-targeted DCs could promote IL-3 expression by CD4 + T cells. Human TSLP-activated DCs are known to express OX40L, which promotes inflammatory Th2 cell responses [26] . Indeed, we found that DCs purified from EDLN of MC903-treated WT mice at D3 exhibited a significant induction of OX40L expression ( Fig. 7a ), together with an increase in the number of CD4 + T cells expressing OX40 (the receptor of OX40L) ( Supplementary Fig. S3 ). Expression of the costimulatory molecules CD80 and CD86 also exhibited a tendency to increase, whereas that of CD40, IL-12p35, IL-12/IL-23p40 and IL-23p19 remained unchanged ( Fig. 7a ). 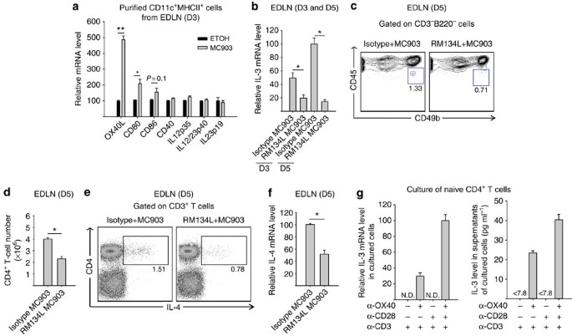Figure 7: A functional axis of OX40L IL-3 in TSLP-promoted Th2 priming. (a) Quantitative RT–PCR analysis of costimulatory molecules and cytokines in purified DCs (CD11c+MHCII+) from ear-draining lymph nodes (EDLN) of MC903- or ETOH-treated wild-type (WT) Balb/c mice at D3. (b–f)In vivoblockade of OX40L using blocking antibody RM134L inhibits TSLP-promoted IL-3 expression, basophil recruitment and Th2 priming. Comparison of IL-3 mRNA levels (b), frequency of basophils (c), CD4+T-cell numbers (d), frequency of IL-4+CD4+T cells (e), and relative IL-4 mRNA level (f) in EDLN from isotype- or RM134L-injected WT Balb/c mice, upon MC903 treatment at D3 or D5 as indicated. (g) Activation of OX40 signal induces IL-3 expression in thein vitrocultured naive CD4+T cells. Naive CD4+T cells isolated from WT spleen were cultured in the presence (+) or absence (−) of agonistic OX40 antibody (α-OX40), combined with the polyclonal stimulation of anti-CD3 (α-CD3) or α-CD3/α-CD28. Left panel, relative IL-3 mRNA level in CD4+T cells at 24 h after culture. Right panel, IL-3 protein level in supernatant of cultured cells at 72 h after culture. ND, not detected. *P<0.05, **P<0.01 (student’st-test). Values are mean±s.e.m. (n≥3). Data are representative of two independent experiments with similar results. Figure 7: A functional axis of OX40L IL-3 in TSLP-promoted Th2 priming. ( a ) Quantitative RT–PCR analysis of costimulatory molecules and cytokines in purified DCs (CD11c + MHCII + ) from ear-draining lymph nodes (EDLN) of MC903- or ETOH-treated wild-type (WT) Balb/c mice at D3. ( b – f ) In vivo blockade of OX40L using blocking antibody RM134L inhibits TSLP-promoted IL-3 expression, basophil recruitment and Th2 priming. Comparison of IL-3 mRNA levels ( b ), frequency of basophils ( c ), CD4 + T-cell numbers ( d ), frequency of IL-4 + CD4 + T cells ( e ), and relative IL-4 mRNA level ( f ) in EDLN from isotype- or RM134L-injected WT Balb/c mice, upon MC903 treatment at D3 or D5 as indicated. ( g ) Activation of OX40 signal induces IL-3 expression in the in vitro cultured naive CD4 + T cells. Naive CD4 + T cells isolated from WT spleen were cultured in the presence (+) or absence (−) of agonistic OX40 antibody (α-OX40), combined with the polyclonal stimulation of anti-CD3 (α-CD3) or α-CD3/α-CD28. Left panel, relative IL-3 mRNA level in CD4 + T cells at 24 h after culture. Right panel, IL-3 protein level in supernatant of cultured cells at 72 h after culture. ND, not detected. * P <0.05, ** P <0.01 (student’s t -test). Values are mean±s.e.m. ( n ≥3). Data are representative of two independent experiments with similar results. Full size image To investigate whether OX40L(DCs)-OX40 (T cells) signalling could mediate IL-3 production in CD4 + T cells, WT mice were i.p. injected with neutralizing anti-OX40L Ab (RM134L) [27] at D0 and D2 during the MC903 treatment. Blockade of OX40L in vivo led to a significant decrease of IL-3 expression in EDLN at both D3 and D5 ( Fig. 7b ); concomitantly, these mice exhibited a significant decrease in basophil recruitment ( Fig. 7c ), CD4 + T-cell expansion ( Fig. 7d ) and IL-4 priming in CD4 + T cells ( Fig. 7e,f ) at D5. To further explore the potential direct effect of OX40L-OX40 signalling on IL-3 expression in naive CD4 + T cells, we employed an in vitro culture system, in which mouse naive CD4 + T cells (CD3 + CD4 + CD62L + ) were cultured in the presence of polyclonal stimulation of anti-CD3 or anti-CD3/anti-CD28. In both cases, activation of the OX40 signal by an agonist anti-OX40 Ab [27] induced IL-3 production, at both mRNA and protein levels ( Fig. 7g ). Taken together, these in vivo and in vitro data demonstrated that TSLP-triggered OX40L-OX40 signalling promoted IL-3 production by naive CD4 + T cells. Employing a topical MC903 treatment to induce TSLP expression in mouse skin KCs, we have dissected the cellular network and signal axis underlying how TSLP drives the initiation of Th2 immune responses in vivo . Our data demonstrate that TSLP-promoted IL-4 initiation in CD4 + T cells of skin-draining LNs involves an orchestrated ‘DC-T-Baso-T’ cascade. Moreover, our results reveal that TSLP-activated DCs first prime naive CD4 + T cells to produce IL-3 through OX40L-OX40 signalling. Subsequently, IL-3 mediates the recruitment of basophils, and basophils in turn promote IL-4 priming in CD4 + T cells. Moreover, IL-3 has an additional role in the optimal expansion of CD4 + T cells, in which basophils are not implicated. These are schematically presented in Fig. 8 and further discussed below. 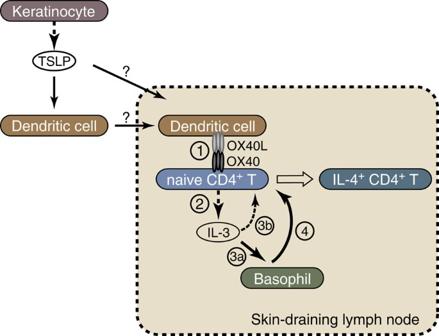Figure 8: A schematic representation of how skin TSLP initiates Th2 responses through an orchestrated DC-T-Baso-T cascade. In the skin-draining lymph nodes (LNs), TSLP-targeted dendritic cells (DCs) activate naive CD4+T cellsviathe OX40L-OX40 signalling (1), thus inducing the production of IL-3 (2). IL-3 mediates the recruitment (and possibly also the activation) of basophils (3a), and is implicated directly or indirectly in the optimal expansion of the CD4+T cells (3b). In turn, the recruited basophils prime the CD4+T cells (4) to express IL-4. Whether and how TSLP produced by KCs activates dermal DCs and triggers their migration to the skin-draining LNs, or TSLP entering LNs (for example, through lymphatic vessel) acts on LN DCs, remains to be investigated (the question marks). Figure 8: A schematic representation of how skin TSLP initiates Th2 responses through an orchestrated DC-T-Baso-T cascade. In the skin-draining lymph nodes (LNs), TSLP-targeted dendritic cells (DCs) activate naive CD4 + T cells via the OX40L-OX40 signalling ( 1 ), thus inducing the production of IL-3 ( 2 ). IL-3 mediates the recruitment (and possibly also the activation) of basophils ( 3a ), and is implicated directly or indirectly in the optimal expansion of the CD4 + T cells ( 3b ). In turn, the recruited basophils prime the CD4 + T cells ( 4 ) to express IL-4. Whether and how TSLP produced by KCs activates dermal DCs and triggers their migration to the skin-draining LNs, or TSLP entering LNs (for example, through lymphatic vessel) acts on LN DCs, remains to be investigated ( the question marks ). Full size image Although TSLP appears to act on various immune cell types (see reviews [3] , [12] ), for example, TSLP could directly promote IL-4 production in mouse CD4 + T cells in vitro [28] , we demonstrate that, in the in vivo context, it is DCs that have a primary role in the initiation of Th2 response driven by skin TSLP ( Fig. 8 ). Indeed, upon DC depletion, IL-3 induction in CD4 + T cells, basophil recruitment in skin-draining LNs and IL-4 priming are all abolished. Of interest, we find that CD11c hi DCs, instead of epidermal LCs, are involved in TSLP-driven Th2 priming. In keeping with our data, a recent study showed that, ablation of Stat5, a transcriptional factor implicated in TSLP signalling, in CD11c hi DCs but not in LCs, diminished the induction of Th2 contact hypersensitivity [29] . It remains yet to be determined whether TSLP produced by KCs activates dermal CD11c hi DCs and triggers their migration to skin-draining LNs, or TSLP entering the draining LNs (for example, through lymphatic vessel) may activate directly the LN CD11c hi DCs (see Fig. 8 ). Further studies are also required to investigate which subset(s) of skin or LN DCs [30] could be the major factor(s) in TSLP-triggered immune response. Although being the primary factor, DCs are not sufficient for optimal IL-4 priming in CD4 + T cells, as we find that basophils are also crucial. As mentioned before, the role of basophils in Th2 cell differentiation has been highly controversial [23] , [25] , [31] , [32] , [33] , [34] , [35] , [36] (see also reviews [18] , [19] ). One argument has been on approaches of basophil depletion, particularly the possible effects of MAR-1 on other cells than basophils [21] , [23] . We have utilized three different strategies (that is, MAR-1, Ba103 or DT) to deplete basophils and found that all of them led to the abrogation of IL-4 induction in CD4 + T cells, thus unequivocally demonstrating that basophils are crucial for an optimal IL-4 initiation triggered by TSLP. It is notable that, upon a longer treatment of MC903 (until D10), IL-4 (as well as IL-13) level in LNs was significantly lower in basophil-depleted mice compared with WT control, although the induction of these cytokines was not completely abolished ( Supplementary Fig. S4 ). This suggests that, in the absence of basophils, other mechanisms (for example, expansion of CD4 + T cells) may possibly contribute to Th2 differentiation (see discussion below). Nevertheless, the controversial reports on the contribution of basophils in Th2 responses in various mouse models may also reflect different requirement of basophils (and TSLP) in different contexts. One major determinant could be the nature of antigen. For example, studies have reported that certain parasite-associated antigens may by pass the requirement of TSLP [37] , basophils [25] and even IL-4 (refs 14 , 38 ) for generating Th2 responses, whereas we have shown that common protein allergen requires TSLP [39] for developing Th2 sensitization. Our data also add further insights into basophil recruitment and function in draining LNs. First, in contrast to previous reports concluding that either DCs [35] or CD4 + T cells [40] alone were sufficient to promote basophil recruitment to draining LNs, we reveal that TSLP-triggered basophil recruitment into skin-draining LNs is mediated by DC-primed naive CD4 + T cells, and therefore it requires both DCs and CD4 + T cells ( Fig. 8 ). Of great importance, our study uncovers for the first time that TSLP-activated DCs prime CD4 + T cells to produce IL-3 at a stage that precedes the induction of IL-4, and IL-3 in turn recruits basophils. Second, our results show that, in contrast to DCs, basophils are dispensable for promoting CD4 + T-cell expansion. Therefore, although basophils have a role in IL-4 induction in CD4 + T cells, they do not seem to behave like the bona fide APCs (antigen presenting cells) to stimulate T-cell proliferation in the draining LNs. How could basophils contribute to TSLP-triggered IL-4 priming? It is possible that basophils provide an initial source of IL-4, particularly under the IL-3 stimulation [31] , [41] , [42] , [43] , and thereby participate in building up a self-reinforcing IL-4 loop in primed CD4 + T cells [18] . Indeed, we observed that basophils sorted from naive mouse spleens produced higher amount of IL-4 upon the in vitro stimulation of IL-3 (but not of TSLP) ( Supplementary Fig. S5 ). To further address the role of IL-4 from basophils, it will be necessary to generate mice in which IL-4 can be selectively and inducibly ablated in basophils. Of note, although eosinophils or mast cells could also provide an initial source of IL-4 (refs 44 , 45 ), and both have been suggested as direct targets of TSLP (see review [3] ), we found that neither eosinophils nor mast cells contributed to TSLP-driven IL-4 initiation because the depletion of either eosinophils (Δdbl GATA mice [46] ) or mast cells (Kit wsh/wsh mice [47] ) did not affect IL-4 induction ( Supplementary Fig. S6 ). Nevertheless, besides IL-4, whether basophils may provide other factor(s) for priming CD4 + T cells and whether such a process implicates a direct contact or a close location between basophils and CD4 + T cells remains still to be clarified. Our analyses identify the OX40L-IL-3 axis in the initiation of Th2 response ( Fig. 8 ). Upon TSLP induction in skin, elevated levels of OX40L and OX40 were seen in LN DCs ( Fig. 7a ) and CD4 + T cells ( Supplementary Fig. S3 ), respectively. Indeed, the OX40L-OX40 signalling has been implicated in T-cell-mediated immunity, for example, through regulating the expansion, survival and effector function of T cells [27] , and has been suggested to have an important role for TSLP-triggered Th2 polarization [26] or TSLP-mediated Th2 lung inflammation [11] . By in vivo OX40L blocking ( Fig. 7b-f ) or in vitro OX40 activation ( Fig. 7g ), we demonstrate for the first time that OX40L-OX40 signalling induces IL-3 expression in naive CD4 + T cells during the Th2 initiation process, although a possible link between IL-3 expression to OX40 signal has been suggested [48] , [49] . Interestingly, this is in contrast to the cytokine IL-2, as the expression of IL-2 was not induced upon the OX40 activation ( Supplementary Fig. S7 ), which is in agreement with a previous study showing that OX40 signalling promoted IL-2 expression in effector but not in naive T cells [50] . The role of IL-3 in Th2 initiation is also of interest. IL-3 has been recognized to be a cytokine produced mainly by activated CD4 + T cells, for example, in response to parasite infection [51] , but little is known about its role in Th differentiation. Importantly, our data indicate that, in TSLP-triggered immune cascade, the induction of IL-3 is prior to IL-4 in CD4 + T cells, and, moreover, IL-3 is critical for IL-4 priming. In addition to its role in mediating basophil recruitment to the skin-draining LNs (see above), IL-3 is also implicated in DC-primed CD4 + T-cell expansion ( Fig.8 ). Indeed, the ablation of IL-3 leads to a significant reduction in CD4 + T-cell expansion ( Fig. 6b,f ), as observed by the blocking of OX40L ( Fig. 7d ), or the depletion of DCs ( Fig. 2f ). These analyses suggest a previously unrecognized function for IL-3 in CD4 + T-cell expansion, besides its better-appreciated role in the development, survival and function of mast cells and basophils [25] , [52] , [53] . How IL-3 has such a role needs to be further explored. Nevertheless, as the expansion of CD4 + T cells does not implicate basophils ( Fig. 3f,l and Supplementary Fig. S1b ), this suggests that, in the absence of basophils, the expansion of CD4 + T cells may contribute to the Th2 cell differentiation probably through autocrine production of IL-4 (ref. 14 ) (see Supplementary Fig. S4 ). In keeping with the mouse in vivo data, human DCs activated by TSLP in vitro also prime naive CD4 + T cells to produce IL-3, notably at an early stage ( Fig. 5f ). Although the in vitro co-culture of TSLP-DCs and CD4 + T cells leads to the increased production of IL-4 (refs 4 , 26 ), we speculate that, in the in vivo context, the presence of basophils would contribute to achieve an optimal and/or earlier Th2 initiation. We are currently underway to establish the in vitro DC-T-basophil co-culture system to explore this speculation and to examine whether the TSLP-OX40L-IL-3 axis has a similar role in the induction of Th2 immune responses in humans. In conclusion, our results in the present study characterize a ‘DC-T-Baso-T’ cellular cascade and reveal OX40L-IL-3 as an important axis in mediating the Th2 priming triggered by skin-derived cytokine TSLP. Further questions are raised. First, do these Th2 initiation mechanisms ( Fig. 8 ) stand in the physiological context(s), and, if yes, in which context(s)? Second, are these Th2 initiation mechanisms specific for TSLP or applied as well to other Th2 promoting cytokines like IL-33 or IL-25; moreover, are they specific for skin or applicable also to other interface barriers including airways or gut epithelia? Notably, it has been recently shown that, in addition to TSLP, IL-25 or IL-33 was capable to promote OX40L in DCs in vitro , and blocking the OX40L signalling diminished Th2 lung inflammation or food allergy [54] . It will be important to functionally validate the implication of OX40L-IL-3 axis in the context of allergy and other diseases related to Th2 immunity [45] , [55] , using pathophysiological animal models and in humans, which may potentially lead to the development of new therapeutic or preventive strategies. Mice Balb/c mice and Rag1 − / − mice (on Balb/c genetic background) were purchased from Charles River Laboratories. Il3 −/− mice [56] were provided by the RIKEN BRC through the National Bio-Resource Project of the MEXT, Japan. Tslp −/− (on Balb/c genetic background) [7] , MCPT8 DTR (on Balb/c genetic background) [22] , Lang-DTREGFP +/− (on Balb/c genetic background) [17] and CD11c-DTR Tg/0 (on C57B6/J genetic background) [15] mice were previously described. Breeding and maintenance of mice were performed under institutional guidelines, and all of the experimental protocols were approved by the animal care and ethic committee of animal experimentation of the Institut de Génétique et de Biologie Moléculaire et Cellulaire (IGBMC) and Institut Clinique de la Souris (ICS). Antibodies and flow cytometry The following antibodies were used: purified anti-FcγRIII/II (CD32/16; Fc Block; clone 2.4G2, (1:50)), FITC-conjugated anti-Gr1 (clone RB6-8C5, (1:100)), PE-conjugated anti-siglec-F (clone E50-2440, (1:50)), V500-conjugated anti-CD3 (clone 500-A2, (1:25)), PerCP-Cy5.5-conjugated anti-CD19 (clone1D3, (1:25)), biotin-conjugated anti-CD4 (clone GK1.5, (1:50)), PerCP-Cy5.5-conjugated anti-CD8a (clone 53-6.7, (1:25)), APC-conjugated anti-IL-4 (clone 11B11, (1:25)) and biotin-conjugated anti-CD11c (clone HL3, (1:50)) were from BD Biosciences; biotin-conjugated anti-CD49b (clone DX5, (1:50)), Alexa700-conjugated anti-CD8a (clone 53-6.7, (1:25)) and FITC-conjugated MHCII (clone M5/114.15.2, (1:50)) were from eBioscience; APC-Cy7-conjugated anti-CD117 (c-kit; clone 2B8, (1:25)), PE-Cy7-conjugated anti-FCεRIα (clone MAR-1, (1:25)), PE-conjugated anti-IL-3 (clone MP2-8F8, (1:25)) and PerCP-Cy5.5- or PE-Cy7-conjugated anti-CD45R (B220; clone RA3-6B2, (1:50)) were from Biolegend; Qdot-585-conjugated streptavidin (1:50) was from Invitrogen; and PE-conjugated streptavidin (1:100) was from Jackson ImmunoResearch. For surface marker staining, ear-draining lymph node (EDLN) cells were incubated with an anti-FcγRII/III Ab (2.4G2) on ice for 10 min to block Fc receptors, washed and incubated with a mix of antibodies on ice for 10 min. Finally, cells were washed and analysed. For intracellular staining, EDLN cells were stimulated for 5 h at 5 × 10 6 cells per ml in the presence of PMA (50 ng ml −1 ; Sigma), ionomycin (500 ng ml −1 ; Sigma) and BD GolgiStop (BD Biosciences). After washing, cells were incubated with anti-FcγRII/III Ab (2.4G2), followed by surface staining for CD3, CD8 and CD4. Cells were then fixed and permeabilized using the BD Cytofix/Cytoperm Kit (BD Biosciences) and stained with anti-IL-4 or anti-IL-3 antibodies. Stained cells were analysed on a LSRII flow cytometer (BD Biosciences). Results were analysed using FlowJo (Treestar). MC903 topical treatment MC903 (calcipotriol; Leo Pharma, Denmark) was dissolved in ethanol (ETOH) and topically applied on mouse ears (1 nmol in 25 μl per ear). As vehicle control, the same volume of ETOH was applied. RNA extraction and quantitative RT–PCR RNA was extracted using TRI Reagent (Sigma-Aldrich) or the RNeasy micro kit (Qiagen). RNA was reverse transcribed using random oligonucleotide hexamers and amplified by quantitative PCR with a Ligthcycler 480 (Roche Diagnostics) and the QuantiTect SYBR Green kit (Qiagen), according to the manufacturer’s instructions. Relative RNA levels were calculated using hypoxanthine phosphoribosyltransferase (HPRT) as internal control. For the analyses of each set of IL-4 or IL-3 expression, an arbitrary unit of 100 was given to the samples with the highest level, and the remaining samples were plotted relative to this value. For the analyses of OX40L, CD80, CD86, CD40, IL-12p35, IL12/23p40, IL-23p19, levels from ETOH-treated samples were set as 100. Sequences of PCR primers are provided in Table 1 (as reported [39] ). Table 1 Sequences of PCR primers. Full size table Isolation of DCs and CD4 + cells from lymph nodes For DCs isolation, LNs were chopped and digested in 2 mg ml −1 collagenase D (Roche), 2.5% FCS and 100 U ml −1 DNAse I (Roche) in PBS at 37 °C for 30 min and then filtered through a 70-μm cell strainer (BD). Single-cell suspensions were incubated with Fc block (FcγRII/III m Ab 2.4G2) for 10 min, and DCs were enriched using CD11c Microbeads (Miltenyi Biotec). CD11c + MHCII + cells were then sorted with FACS Aria II (BD) (purity was>95%). For CD4 + cell isolation, EDLN were chopped and mechanically disrupted and then filtered through a 70-μm cell strainer. CD4 + cells were isolated using CD4 + T-cell isolation kit II (Miltenyi Biotec) (purity was >95%). Depletion of DCs or Langerhans cells in mice For depletion of CD11c hi DCs, CD11c-DTR Tg/0 mice [15] were injected i.p. with diphtheria toxin (DT) (100 ng per 25 g body weight) at D -1 (that is, one day before MC903 or ETOH treatment). DT-injected CD11c-DTR 0/0 littermate mice were used as controls. For depletion of Langerhans cells, Lang-DTREGFP +/− mice [17] received an i.p. injection of DT (1 μg per 25 g body weight) at D -1. The DT-injected wild-type littermate mice were used as controls. These mice were then treated with MC903 or ETOH at D0, D2 and D4, as indicated. Basophil depletion in mice For antibody-mediated depletion of basophils, wild-type Balb/c mice were injected i.p. twice daily for 3 days from D -4 (that is, four days before MC903 or ETOH treatment) to D -2 (that is, two days before MC903 or ETOH treatment) with 5 μg of Armenian hamster-anti-mouse FcεRIα (clone MAR-1, eBioscience) or injected i.v. with 30 μg of rat-anti-mouse CD200R3 (clone Ba103, Hycult Biotech) at D -2. For DT-mediated depletion of basophils, MCPT8 DTR mice (in Balb/c genetic background) received an i.p. injection of DT (750 ng per 20 g body weight) at D -2. These mice were then treated with MC903 or ETOH at D0, D2 and D4, as indicated. Adoptive transfer of CD4 + T cells CD4 + T cells were purified from spleens of wild-type Balb/c or Il3 −/− mice using mouse CD4 + T-cell Isolation Kit II (Miltenyi) and were intravenously ( i.v. ) injected (5 × 10 6 cells) to Rag1 −/− recipient mice 24 h before MC903 treatment. Naive T-cell culture Naive CD4 + T cells from spleens of wild-type Balb/c mice were isolated using the CD4 + CD62L + T-cell isolation kit II (Miltenyi Biotec), following the manufacturer’s instructions. Purified naive T cells (1 × 10 6 per ml) were cultured in anti-CD3 (2 μg ml −1 ; clone 145-2C11, eBioscience)-coated wells either in the presence or absence of the anti-CD28 (2 μg ml −1 ; clone 37–51, eBioscience) antibody in RPMI 1640 medium supplemented with 10% of FCS and 2 mM of L -glutamine. To activate OX40 signalling, agonistic rat-anti-mouse OX40 Ab (5 μg ml −1 ; clone OX86, Biolegend) was added to the culture. Cells and supernatants were collected for RT–PCR or ELISA analyses. IL-3 protein levels in culture supernatants were measured using the mouse IL-3 Quantikine ELISA kit (R&D) (the detection limit was 7.8 pg ml −1 ). In vivo blockade of OX40L To block OX40L–OX40 interaction, mice were injected i.p. with 300 μg of rat anti-mouse-OX40L neutralizing mAb (clone RM134L, rat IgG2bκ, BioXcell) or isotype control antibody IgG2b, given at D0 and D2 at the same time during MC903 skin treatment (see Fig. 1a ). Human DC-naive CD4 + T-cell co-culture Buffy coats were obtained from healthy donors (Saint-Antoine Crozatier Blood Bank, Paris, France) with informed consent for research use in accordance with the declaration of Helsinki. CD11c + DC were isolated from peripheral blood mononuclear cells by using the Easy Sep human pan-DC pre-enrichment kit (Stem Cell) followed by cell sorting to lineage − CD11c + cells by flow cytometry (purity was >99%). Naive CD4 + T cells (CD4 + CD25 − CD45RA + CD45RO − ) were purified from healthy donors as previously described [57] , [58] . DCs were seeded in 96-well flat-bottom plates in medium alone or in presence of human TSLP (50 ng ml −1 ; R&D). Twenty-four hours after, DCs were washed and co-cultured with naive CD4 + T cells in complete Yssel medium at a ratio of 1:5. After 1, 2, 3, 4 or 5 days, cells were washed and re-stimulated with anti-human CD3/CD28-coupled microbeads (Invitrogen) for 24 h as described [58] . Supernatants were collected and assayed for IL-3 and IL-4 levels using cytometric bead assay Flex Sets (BD Biosciences; detection limit was 20 pg ml −1 for both). Statistical analysis Data were analysed using SigmaStat (Systat Software, Point Richmond, CA, USA) by Student’s t -test or the Mann–Whitney rank sum nonparametric test depending on results from the Kolmogorov–Smirnov test (with Lilliefors’ correction) for normality and Levene Median test for equal variance. How to cite this article: Leyva-Castillo, J.M. et al. Skin thymic stromal lymphopoietin initiates Th2 responses through an orchestrated immune cascade. Nat. Commun. 4:2847 doi: 10.1038/ncomms3847 (2013).